Interactions between Twist and other core epithelial–mesenchymal transition factors are controlled by GSK3-mediated phosphorylation A subset of transcription factors classified as neural crest ‘specifiers’ are also core epithelial–mesenchymal transition regulatory factors, both in the neural crest and in tumour progression. The bHLH factor Twist is among the least well studied of these factors. Here we demonstrate that Twist is required for cranial neural crest formation and fate determination in Xenopus . We further show that Twist function in the neural crest is dependent upon its carboxy-terminal WR domain. The WR domain mediates physical interactions between Twist and other core epithelial–mesenchymal transition factors, including Snail1 and Snail2, which are essential for proper function. Interaction with Snail1/2, and Twist function more generally, is regulated by GSK-3-β-mediated phosphorylation of conserved sites in the WR domain. Together, these findings elucidate a mechanism for coordinated control of a group of structurally diverse factors that function as a regulatory unit in both developmental and pathological epithelial–mesenchymal transitions. The neural crest (NC) is a proliferative, multipotent stem cell population that arises at the neural plate border (NPB) during mid-gastrulation, and ultimately gives rise to diverse derivatives that include neurons and glia of the peripheral nervous system, facial cartilage/bone and melanocytes [1] , [2] . NC cells undergo an epithelial–mesenchymal transition (EMT), delaminate from the neuroepithelium and migrate to diverse sites throughout the embryo where they will differentiate [1] , [2] , [3] , [4] , [5] . NC cells retain multipotency until early migratory stages via a mechanism dependent upon c-myc and Id3 [6] , [7] , before becoming competent to respond to signals that will induce differentiation. NC formation is one of the few examples during embryonic development where a newly induced cell type exhibits greater developmental potential than the cells from which it was derived, making the NC a fascinating model for asking questions about the molecular underpinnings of ‘stemness’ and its relationship to the capacity for migratory/invasive cell behaviour. In response to NC-inducing signals, cells at the NPB initiate expression of NC ‘specifier’ genes, including Snail family members Snail1 and Snail2 (also known as Slug ), SoxE factors ( Sox8 , 9 and 10 ), the WH factor Foxd3 and the bHLH factor Twist [3] , [8] , [9] , [10] , [11] , [12] , [13] , [14] , [15] , [16] , [17] , [18] , [19] , [20] , [21] , [22] . Collectively, these diverse factors constitute a gene regulatory network (GRN) that governs formation and maintenance of the NC precursor population [17] , [18] , [19] . A subset of the proteins that control formation of NC stem cells are used reiteratively to control the subsequent EMT and migratory behaviour of NC cells [19] , [23] . Importantly, these same factors, including Snail1, Snail2 and Twist, are core EMT regulatory factors and are also deployed during tumour progression, and in other developmental contexts, to control this complex cellular transition [5] , [19] , [20] , [21] , [24] . Snail1 and Snail2 are the best-studied transcriptional regulators involved in both NC specification and EMT [2] , [17] , [18] , [19] , [20] , [21] , [23] , [24] . These zinc-finger repressors are essential for formation of NC stem cells as well as for the onset of NC migration, and can directly downregulate genes involved in cell adhesion and junctions [22] , [25] , [26] , [27] , [28] . Importantly, while Snail proteins can potently induce EMTs, their ability to drive this transition is highly context dependent. For example, Snail factors direct formation of NC stem cells many hours before those cells will become migratory [23] . Similarly, Snail factors are expressed at the NPB in non-vertebrate chordates in cells that never become migratory [29] . Thus, cellular context dictates when Snail proteins promote ‘stemness’ versus migratory/invasive behaviour. Recent work has indicated that cellular levels of Snail proteins are one key determinant of their functional output during NC cell development [30] . Snail1/2 protein levels are regulated by the ubiquitin–proteasome system (UPS), and these proteins are targeted for proteasomal degradation by the F-box protein Partner of paired (Ppa, also known as FBXL14). Stabilized Snail proteins that cannot be targeted by Ppa induce premature NC migration [30] , demonstrating the necessity of tightly regulating the threshold levels of these factors present in cells. It is likely, however, that additional mechanisms also contribute to controlling Snail protein function in a context-dependent manner. The bHLH factor Twist has been classified as a NC specifier [17] , [18] , [19] , although it does not appear to have this role in amniotes. Importantly, like Snail1/2, Twist also functions as a core EMT regulatory factor in both developmental and pathological contexts [31] . Twist possesses a basic domain that can interact with core Ebox sequence ‘CANNTG,’ a helix–loop–helix (HLH) domain that mediates homodimerization or dimerization with E12/E47, and a highly conserved C-terminal domain, the WR domain or Twist box [32] . The WR domain has been shown to physically interact with another non-bHLH transcription factor, Runx2, to inhibit osteoblast-specific gene expression [33] , and recently has been shown to similarly inhibit Sox9 activity during chondrogenesis [34] . It has also been suggested that the WR domain can function as an activation domain for Twist-E12 dimers [35] . More recently, it has been shown that Twist, like Snail family proteins, is targeted for UPS-mediated degradation by the F-box protein Ppa, and this regulation is dependent upon the WR domain [36] . Twist is implicated in the EMT/progression of multiple epithelial cancers, and its expression correlates with invasiveness and poor outcome [5] , [37] , [38] , [39] , [40] . Twist can also promote increased cell proliferation and the ability to evade apoptosis in aggressive tumour cells [37] , [41] , [42] . Expression of this factor in primary tumour cells has been shown to override oncogene-induced cellular senescence and apoptosis [43] , [44] , [45] , and has been linked to the maintenance of a ‘cancer stem cell’ state [46] , [47] , [48] . Twist is distinguished from other NC specifiers by the restriction of its expression to cranial regions. This localization suggests that Twist might have a role in endowing cranial NC precursors with the ability to give rise to mesectodermal derivatives, such as cartilage and bone. A better understanding of the function and regulation of Twist is essential to understanding NC stem cell formation and the EMT/migration of these cells, and will shed important light on Twist’s role in regulating related states during tumour formation and metastasis. Here, using Xenopus as a model, we examine the expression and function of Twist in NC crest formation in cranial regions. We find that both gain and loss of Twist expression is incompatible with normal NC development in Xenopus , indicating that correct levels of Twist expression are key to its function, and suggesting that this factor may be regulated, at least in part, by protein–protein interactions. Consistent with such a model, we show that Twist physically interacts with core EMT factors Snail1 and Snail2 through its conserved WR domain, and inhibits the NC-inducing activity of these factors. Finally, we identify multiple GSK3-β phosphorylation sites in the Twist C-terminus, and show that phosphorylation of these sites is essential for Twist function and for its inhibitory interactions with Snail proteins. Our results lend important regulatory insights into a factor that has key roles in both development and cancer. Twist is expressed in premigratory and migratory NC cells In Xenopus , the expression of a number of NC ‘specifiers’, including Snail1 , Snail2 , Sox8 , Sox9 and Foxd3 , can be detected at the NPB by late gastrula stages (Nieuwkoop and Faber stages 11.5–12). These factors are expressed throughout all NC precursors regardless of axial level [19] , [21] . Twist expression is distinct from other NC specifiers both temporally and spatially. Twist expression is first detectable in NC precursor cells at stage 14, considerably later than several other NC specifiers, including Snail1 , Snail2 , Sox9 and Foxd3 , indicating that it is unlikely to be a regulatory input into the initial expression of these factors. Twist expression initiates in an anterior to posterior progression, beginning in the presumptive mandibular crest ( Fig. 1a ) and subsequently expanding to the hyoid and then branchial NC segments. Importantly, unlike other NC specifiers, Twist expression remains restricted to cranial regions and is not found in NC cells posterior to the branchial NC segment. Twist is maintained in cranial NC cells as they commence migration ventrally into the pharyngeal pouches, a period when they retain stem cell attributes, and is maintained in NC in the branchial arches through post-migratory stages ( Supplementary Fig. S1 ). 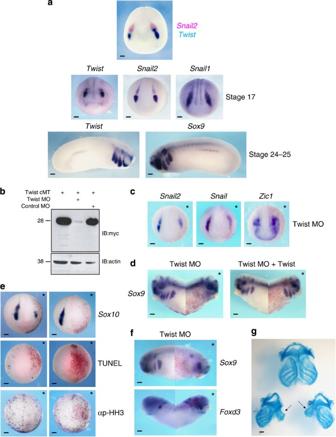Figure 1: Twist is required for NC development. (a) Top: doublein situcomparingSnail2expression (magenta) toTwist(light blue, dark blue in overlap). Middle:in situcomparing expression ofTwist,Snail1andSnail2at stage 17. Bottom:in situcomparingTwistandSox9expression at stages 24–25. Demonstrating that the onset ofSnail2expression in posterior cranial regions (mandibular and branchial) precedesTwistand that expression of Twist in the neural crest is restricted to cranial regions. (b) Western blot demonstrating efficient depletion of Twist (C-terminal myc-epitope-tagged cMT) protein in the presence of Twist MO but not control MO in blastula-stagedXenopusembryos (stage 9). (c)In situhybridization of Twist MO-injected embryos at stage 16.Snail1,Snail2expression is diminished whileZic1is enhanced. (d) Stage 28 embryos were injected with Twist MO alone, or Twist MO and a form of Twist unable to be targeted by the MO.Sox9expression is rescued by co-injection of Twist demonstrating the specificity of the MO effects. (e) Top:in situhybridization of Twist MO-injected embryos at stage 17 showing loss ofSox10expression. Middle: Twist MO does not alter the numbers of TUNEL-positive cells. Bottom: Twist MO does not alter levels of cell proliferation as visualized by phosphohistone H3 immunostaining. (f) MO-mediated Twist depletion inXenopusembryos at stage 28 were examined viain situhybridization analysing the cartilage marker,Sox9, and the glial cell marker,Foxd3. Twist depletion inhibitsSox9and increasesFoxd3. (g) Alcian Blue staining examining cranial cartilage formation in control (Top) or Twist MO (Bottom). Arrows indicated injected side (stage 40–43). β-galactosidase staining (in red) and asterisk marks manipulated side of the embryos in panelsc–f. Scale bars, 200 μm. IB, immunoblotting. Figure 1: Twist is required for NC development. ( a ) Top: double in situ comparing Snail2 expression (magenta) to Twist (light blue, dark blue in overlap). Middle: in situ comparing expression of Twist , Snail1 and Snail2 at stage 17. Bottom: in situ comparing Twist and Sox9 expression at stages 24–25. Demonstrating that the onset of Snail2 expression in posterior cranial regions (mandibular and branchial) precedes Twist and that expression of Twist in the neural crest is restricted to cranial regions. ( b ) Western blot demonstrating efficient depletion of Twist (C-terminal myc-epitope-tagged cMT) protein in the presence of Twist MO but not control MO in blastula-staged Xenopus embryos (stage 9). ( c ) In situ hybridization of Twist MO-injected embryos at stage 16. Snail1 , Snail2 expression is diminished while Zic1 is enhanced. ( d ) Stage 28 embryos were injected with Twist MO alone, or Twist MO and a form of Twist unable to be targeted by the MO. Sox9 expression is rescued by co-injection of Twist demonstrating the specificity of the MO effects. ( e ) Top: in situ hybridization of Twist MO-injected embryos at stage 17 showing loss of Sox10 expression. Middle: Twist MO does not alter the numbers of TUNEL-positive cells. Bottom: Twist MO does not alter levels of cell proliferation as visualized by phosphohistone H3 immunostaining. ( f ) MO-mediated Twist depletion in Xenopus embryos at stage 28 were examined via in situ hybridization analysing the cartilage marker, Sox9 , and the glial cell marker, Foxd3 . Twist depletion inhibits Sox9 and increases Foxd3 . ( g ) Alcian Blue staining examining cranial cartilage formation in control (Top) or Twist MO (Bottom). Arrows indicated injected side (stage 40–43). β-galactosidase staining (in red) and asterisk marks manipulated side of the embryos in panels c – f . Scale bars, 200 μm. IB, immunoblotting. Full size image Twist is required for normal NC development As Twist is expressed in NC precursors and has been categorized in the context of the NC-GRN as a ‘neural crest specifier’, we investigated the consequences of loss of Twist function for NC development. A translation blocking morpholino (MO) that can deplete Twist protein from early embryos ( Fig. 1b ) was injected, together with β-galactosidase as a lineage tracer, in one cell at the 8-cell stage to target NC and avoid effects on the mesoderm (where Twist is also expressed). Embryos were cultured to early neurula stages and examined for expression of components of the NC-GRN ( Fig. 1c ). NC-GRN factors whose expression precedes that of Twist in NC cells, such as Snail1 , Snail2 ( Fig. 1c ), were inhibited but less affected by Twist depletion than was Sox10 , which has a later onset of expression ( Fig. 1e ). In contrast to the loss of NC specifier expression, we found that expression domain of Zic1 , a NPB specifier [17] , [18] , [19] , was expanded in Twist-depleted embryos, suggesting that the cells that did not express NC markers were stalled in a NPB state and/or adopted alternative fates, such as placodes ( Fig. 1c ). Importantly, the effects of Twist depletion can be rescued by a form of Twist that cannot be targeted by the MO ( Fig. 1d ). As the expression of a number of NC specifiers was diminished following Twist depletion, we examined whether their loss could be attributed to an increase in the number of apoptotic cells. Embryos injected with Twist MO were allowed to develop to mid-neurula stages (stage 17) when apoptosis was assessed by TdT-mediated dUTP nick end labelling (TUNEL) staining. Only a few TUNEL-positive nuclei were observed on both Twist-depleted and control sides of these embryos ( Fig. 1e ), strongly suggesting that the loss of gene expression reflects altered cell specification as opposed to the death of specific cell populations. Similarly, we asked if observed changes in gene expression could be a consequence of altered cell proliferation/cell cycle progression by examining the numbers of cells immunoreactive for phosphohistone H3. Again, no difference was noted in numbers of mitotic cells on the Twist-depleted versus control sides of the embryos. Loss of Twist alters NC fate diversification Given that not all NC gene expression was lost in Twist-depleted embryos, we examined the consequences of Twist depletion for formation of cranial NC derivatives to gain insights into the role of Twist in NC fate diversification in Xenopus . Accordingly, embryos injected with Twist MO at the 8-cell stage were cultured to stages where effects on NC derivatives could be evaluated. At stage 28, injected embryos exhibited reduced expression of Sox9 in the branchial arches, where it marks developing chondrocytes ( Fig. 1f ) and by stage 43 profound defects in cartilage formation and morphogenesis were observed ( Fig. 1g ). Conversely, Foxd3 , which is expressed in presumptive cranial glial cells at stage 28, was increased ( Fig. 1f ), suggesting that in the absence of Twist, cranial NC cells that would normally give rise to cartilage might instead adopt glial fates. Twist misexpression interferes with NCC development We further probed the function of Twist in NC cells through gain-of-function experiments. Twist misexpression led to increased Snail1 expression, whereas expression of Snail2 and Sox10 was diminished ( Fig. 2a ). These changes in NC gene expression were not owing to changes in proliferation or the numbers of apoptotic cells ( Fig. 2b ). As Twist depletion in cranial NC precursors had profound consequences for NC fate diversification, we asked if Twist misexpression would as well. Significantly, Twist misexpression caused defects opposite to those observed in Twist-depleted embryos. Expression of Sox9 in the branchial arches was enhanced, whereas expression of Foxd3 was greatly diminished ( Fig. 2c ). 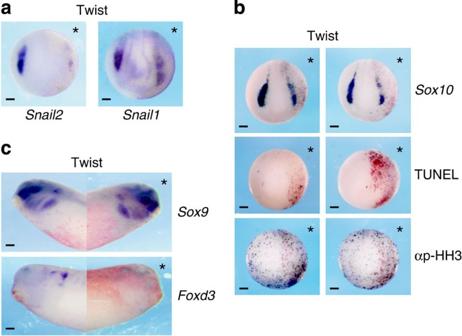Figure 2: Misexpression of Twist interferes with neural crest development. (a)In situhybridization of stage 16/17 embryos expressing exogenous Twist. Twist decreasesSnail2expression in premigratory NC cells but can increaseSnail1expression. (b)Xenopusembryos misexpressing Twist were examined at stage 17 for changes in cell death (TUNEL staining) or cell proliferation (α-phospho histone H3 staining). Top:Sox10is downregulated in response to Twist misexpression. Middle: Twist misexpression does not lead to increased TUNEL staining. Bottom: Twist misexpression does not alter the numbers of cells immunoreactive for phosphohistone H3. (c) Embryos expressing ectopic Twist were examined viain situhybridization at stage 28 analysing the cartilage marker,Sox9, and the glial cell marker,Foxd3. Twist increasesSox9and inhibitsFoxd3expression. β-galactosidase staining (in red) and asterisk marks manipulated side of the embryos in panelsa–c. Scale bars, 200 μm. Figure 2: Misexpression of Twist interferes with neural crest development. ( a ) In situ hybridization of stage 16/17 embryos expressing exogenous Twist. Twist decreases Snail2 expression in premigratory NC cells but can increase Snail1 expression. ( b ) Xenopus embryos misexpressing Twist were examined at stage 17 for changes in cell death (TUNEL staining) or cell proliferation (α-phospho histone H3 staining). Top: Sox10 is downregulated in response to Twist misexpression. Middle: Twist misexpression does not lead to increased TUNEL staining. Bottom: Twist misexpression does not alter the numbers of cells immunoreactive for phosphohistone H3. ( c ) Embryos expressing ectopic Twist were examined via in situ hybridization at stage 28 analysing the cartilage marker, Sox9 , and the glial cell marker, Foxd3 . Twist increases Sox9 and inhibits Foxd3 expression. β-galactosidase staining (in red) and asterisk marks manipulated side of the embryos in panels a – c . Scale bars, 200 μm. Full size image Twist interacts with core EMT factors Snail1 and Snail2 It was notable that Twist depletion and misexpression had similar consequences for the expression of some early NC factors (for example, Snail2 and Sox10 ). Similar phenotypes in gain- and loss-of-function experiments can indicate functional dependence on protein–protein interactions, where proper stoichiometry is essential. As Twist helps maintain osteoblast precursors in an undifferentiated state by binding and inhibiting Runx2 (ref. 33 ), we asked if Twist might bind to, and modulate the activity of, other NC regulatory factors. Embryos co-expressing myc-tagged Twist protein and flag-tagged forms of NC regulatory proteins Snail1, Snail2, Ppa and LMO4 were cultured to late blastula stages when putative interacting factors were immunoprecipitated and their ability to bind Twist evaluated by western blot. Twist displayed robust interactions with both Snail1 and Snail2 ( Fig. 3a ), indicating that its function in cranial NC cells may be at least partially dependent upon its ability to interact with other core EMT factors. By contrast, Twist was unable to interact with LMO4, a Snail1/2-binding LIM adaptor protein essential for NC formation [49] . Interaction between Snail2 and Twist was found to depend mainly upon the Snail2 C-terminus, and does not require the SNAG domain ( Fig. 3b ). 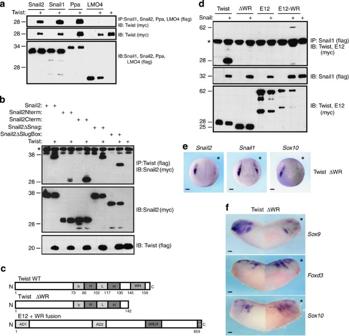Figure 3: Twist physically interacts with core EMT factors Snail1 and Snail2 through its WR domain. (a) Western blot showing co-IP of myc-tagged Twist from embryo lysates co-expressing Flag-tagged neural crest regulatory factors Snail1, Snail2, Ppa and LMO4. Strong interaction with both Snail1 and Snail2 but not LMO4 is observed. Ppa serves as a positive control. (b) Co-Immunoprecipitation of myc-tagged Twist from embryo lysates co-expressing myc-tagged Snail2 isoforms (wild-type, Nterm, Cterm, ΔSnag or ΔSlug box). Interaction with the Snail2 C-terminus is significantly stronger than with the amino-terminus and interaction does not require the SNAG domain, IgG bands indicated by asterisk. (c) Schematic illustrating the Twist deletion and E12–WR fusion constructs used in experiments. AD denotes the activation domains within E12 protein. (d) Western blot showing IP of Snail1 from embryo lysates co-expressing WT Twist, Twist ΔWR, E12 or E12+ ΔWR. Deletion of the WR domain abolishes Twist interaction with Snail1. E12 does not interact with Snail1, whereas the fusion protein does interact. IgG bands are indicated by an asterisk. (e)In situhybridization ofXenopusembryos misexpressing Twist ΔWR RNA during premigratory neural crest stages (stages 16–17). Twist ΔWR decreasesSnail1,Snail2andSox10expression. (f)Xenopusembryos injected with Twist ΔWR were examined at stage 28 viain situhybridization for expression of the cartilage marker,Sox9, and the glial cell markers,Foxd3andSox10. Deletion of the WR domain inhibitsSox9and increasesSox10andFoxd3expression. β-galactosidase staining (in red) and asterisk marks manipulated side of the embryo. Scale bars, 200 μm. IB, immunoblotting. Figure 3: Twist physically interacts with core EMT factors Snail1 and Snail2 through its WR domain. ( a ) Western blot showing co-IP of myc-tagged Twist from embryo lysates co-expressing Flag-tagged neural crest regulatory factors Snail1, Snail2, Ppa and LMO4. Strong interaction with both Snail1 and Snail2 but not LMO4 is observed. Ppa serves as a positive control. ( b ) Co-Immunoprecipitation of myc-tagged Twist from embryo lysates co-expressing myc-tagged Snail2 isoforms (wild-type, Nterm, Cterm, ΔSnag or ΔSlug box). Interaction with the Snail2 C-terminus is significantly stronger than with the amino-terminus and interaction does not require the SNAG domain, IgG bands indicated by asterisk. ( c ) Schematic illustrating the Twist deletion and E12–WR fusion constructs used in experiments. AD denotes the activation domains within E12 protein. ( d ) Western blot showing IP of Snail1 from embryo lysates co-expressing WT Twist, Twist ΔWR, E12 or E12+ ΔWR. Deletion of the WR domain abolishes Twist interaction with Snail1. E12 does not interact with Snail1, whereas the fusion protein does interact. IgG bands are indicated by an asterisk. ( e ) In situ hybridization of Xenopus embryos misexpressing Twist ΔWR RNA during premigratory neural crest stages (stages 16–17). Twist ΔWR decreases Snail1 , Snail2 and Sox10 expression. ( f ) Xenopus embryos injected with Twist ΔWR were examined at stage 28 via in situ hybridization for expression of the cartilage marker, Sox9 , and the glial cell markers, Foxd3 and Sox10 . Deletion of the WR domain inhibits Sox9 and increases Sox10 and Foxd3 expression. β-galactosidase staining (in red) and asterisk marks manipulated side of the embryo. Scale bars, 200 μm. IB, immunoblotting. Full size image Twist function requires the C-terminal WR domain In osteoblasts, Twist’s interaction with Runx2 is dependent upon its C-terminal WR domain. We therefore asked if Twist function in the cranial NC required this domain. We generated a Twist isoform with the WR domain deleted (Twist-ΔWR, Fig. 3c ). Co-immunoprecipitation (co-IP) assays comparing Snail binding to WT Twist or Twist-ΔWR demonstrated that the WR domain is necessary for interaction with Snail ( Fig. 3d ). Glutathione S -transferase (GST)-pulldown assays indicate that the interaction between Twist and Snail2 is direct ( Supplementary Fig. S1B ). Consistent with its interaction with the Snail2 C-terminus, Twist diminishes recruitment of Snail2 to chromatin, whereas Twist-ΔWR does not ( Supplementary Fig. S2C,D ). To determine if the WR domain is sufficient to mediate Snail interaction, this peptide was fused to the C-terminus of bHLH protein E12 ( Fig. 3c ), which cannot itself interact with Snail. The E12–WR fusion protein was able to bind Snail, indicating that the WR domain is sufficient to mediate this interaction ( Fig. 3d ). We further asked if the phenotypic consequences of Twist expression in the cranial NC were dependent upon the WR domain. At neural plate stages, Twist-ΔWR expression resulted in loss of Snail1 , Snail2 and Sox10 ( Fig. 3e ), similar to what is observed following Twist depletion ( Fig. 1c ). We also examined the effects of Twist-ΔWR on cranial NC cell fate diversification. Embryos injected with Twist-ΔWR displayed decreased Sox9 expression in the branchial arches ( Fig. 3f ). Conversely, Twist-ΔWR-expressing embryos showed increased expression of both Sox10 and Foxd3 in presumptive cranial glia ( Fig. 3f ). These results phenocopy the effects of Twist depletion ( Fig. 1f ), suggesting that deletion of the WR domain creates a dominant inhibitory form of Twist, at least with respect to roles in NC cell fate diversification. Importantly, Twist-ΔWR does not act as a general inhibitor of bHLH protein function; for example, it does not interfere with the ability of neurogenin to induce ectopic neurogenesis nor does it block Mitf activation of the Dct promoter ( Supplementary Fig. S2A,B ). WR domain mutations alter Twist binding to Snail1/2 A previously characterized mouse Twist mutation known as ‘Charlie Chaplin’ promotes premature osteoblast differentiation [50] and inhibits Twist interaction with Runx2 (ref. 33 ). The causal mutation is a proline substitution in the WR domain. In the WR domain of Xenopus Twist (amino acids (aa) 143–166), this mutation corresponds to Twist S152P . We generated Twist mutants in which serine 152 was substituted either with proline to mimic the ‘Charlie Chaplin’ mutation, or with alanine. In co-IP assays, the proline substitution enhanced interaction with Snail2 whereas the alanine mutation frequently diminished interaction but sometimes had no effect ( Fig. 4a ), suggesting that this site has a role in the interaction but is not the main regulatory site ( Fig. 4a ). Importantly, the sequence proximal to serine 152 includes a serine residue four aa upstream, a spacing characteristic of target sites for GSK-3β, which shows sequence preference for S xxxS* (where ‘x’ is any aa and S* represents a ‘priming’ phosphorylation) ( Fig. 4b ). To determine if serine 148 regulates interaction between Twist and other core EMT factors, this residue was mutated to alanine or aspartic acid. Twist S148A blocked interaction between Twist and Snail2, whereas Twist S148D strongly enhanced interaction ( Fig. 4c ) consistent with a model whereby phosphorylation of Twist at serine 148 regulates protein–protein interactions with the EMT factors Snail1/2. 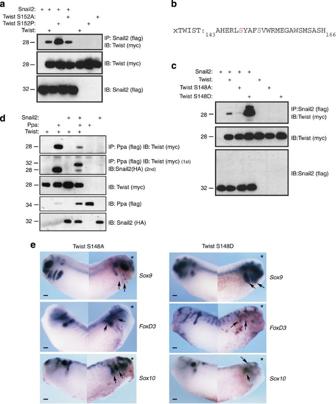Figure 4: Mutations in the WR domain modulate interactions between Twist and core EMT factors. (a) Co-immmunoprecipitation showing that a characterized serine to proline mutation (S152P) in the Twist WR domain enhances interaction with Snail2 whereas mutation of this residue to alanine (S152A) has no effect. (b) Amino-acid sequence of the Twist WR domain highlighting in red (S148) or blue (S152) residues mutated in (a,c,d). (c) Twist serine 148 regulates protein–protein interactions with other core EMT factors, such as Snail2. Mutation of serine 148 to alanine (S148A) inhibits Twist interaction with Snail2 while mutation to aspartate (S148D) significantly enhances Twist interaction with Snail2. Immunoprecipitates were resolved by SDS–PAGE, and Snail2-bound Twist was detected by α-Myc western blotting. (d) Co-IP examining Twist interaction with Ppa in the presence or absence of co-expressed Snail2. Ppa-bound Twist was detected by α-Myc western blotting. Snail2 interferes with the Ppa–Twist interaction. Western blot was then reprobed to visualize Ppa–Snail2 interaction using α-haemagglutinin (HA) western blotting. Snail2 interaction with Ppa is robust despite co-expressed Twist. (e) Embryos expressing Twist S148A or Twist S148D were examined viain situhybridization at stage 28 for expression of cartilage marker,Sox9, and the glial cell markers,Foxd3andSox10. Twist S148A inhibitsSox9expression and leads to enhancedFoxd3andSox10expression whereas Twist S148D enhancesSox9expression and leads to decreased expression ofFoxd3andSox10. Arrows mark the regions where developing cranial ganglia and branchial arch cartilages are affected. β-galactosidase staining (in red) and asterisk marks manipulated side of the embryo. Scale bars, 200 μm. IB, immunoblotting. Figure 4: Mutations in the WR domain modulate interactions between Twist and core EMT factors. ( a ) Co-immmunoprecipitation showing that a characterized serine to proline mutation (S152P) in the Twist WR domain enhances interaction with Snail2 whereas mutation of this residue to alanine (S152A) has no effect. ( b ) Amino-acid sequence of the Twist WR domain highlighting in red (S148) or blue (S152) residues mutated in ( a , c , d ). ( c ) Twist serine 148 regulates protein–protein interactions with other core EMT factors, such as Snail2. Mutation of serine 148 to alanine (S148A) inhibits Twist interaction with Snail2 while mutation to aspartate (S148D) significantly enhances Twist interaction with Snail2. Immunoprecipitates were resolved by SDS–PAGE, and Snail2-bound Twist was detected by α-Myc western blotting. ( d ) Co-IP examining Twist interaction with Ppa in the presence or absence of co-expressed Snail2. Ppa-bound Twist was detected by α-Myc western blotting. Snail2 interferes with the Ppa–Twist interaction. Western blot was then reprobed to visualize Ppa–Snail2 interaction using α-haemagglutinin (HA) western blotting. Snail2 interaction with Ppa is robust despite co-expressed Twist. ( e ) Embryos expressing Twist S148A or Twist S148D were examined via in situ hybridization at stage 28 for expression of cartilage marker, Sox9 , and the glial cell markers, Foxd3 and Sox10 . Twist S148A inhibits Sox9 expression and leads to enhanced Foxd3 and Sox10 expression whereas Twist S148D enhances Sox9 expression and leads to decreased expression of Foxd3 and Sox10 . Arrows mark the regions where developing cranial ganglia and branchial arch cartilages are affected. β-galactosidase staining (in red) and asterisk marks manipulated side of the embryo. Scale bars, 200 μm. IB, immunoblotting. Full size image To determine if serine 148 is essential for Twist function during NC fate diversification, embryos expressing Twist S148A or Twist S148D were examined by in situ hybridization for formation of NC derivatives. Embryos expressing Twist S148A showed decreased expression of Sox9 in the developing branchial arches at stage 28 ( Fig. 4e ), and decreased and malformed facial cartilages at stage 43 ( Supplementary Fig. S3 ). Conversely, Twist S148D -expressing embryos showed increased Sox9 expression, similar to wild-type Twist ( Fig. 2c ). Twist S148A -expressing embryos showed increased expression of both Sox10 and Foxd3 in presumptive cranial glia whereas Twist S148D had the opposite effect. Together, these findings suggest that phosphorylation of Twist at serine 148 is required for normal NC fate diversification. Snail co-expression modulates Twist stability Physical interaction between Snail1/2 and Twist could have many potential functional consequences significant to the regulation of both NC development and developmental/pathological EMTs. As Twist stability is regulated by the UPS and is controlled in part by the WR domain, we asked if co-expression of Snail1 or Snail2 altered Twist stability. Embryos expressing Twist alone, or co-expressing Snail1, were cultured over developmental time and collected at set time intervals for western analysis. Co-expression of Snail1 was found to stabilize Twist ( Supplementary Fig. S3B ). A potential mechanism for this stabilization is provided by the finding that co-expressing Snail2 interferes with the interaction between Twist and Ppa ( Fig. 4d ), suggesting that Snail2 may have greater affinity for Ppa than does Twist. Twist is a substrate for GSK-3β-mediated phosphorylation As serine 148 resembles a GSK-3β site, we used immune-complex kinase assays to determine if Twist could be phosphorylated by GSK-3β in vitro . We noted that there were two additional SxxxS motifs in the Twist C-terminus, up and downstream of serine 148/152, and generated serine to alanine mutations in each of them ( Fig. 5a ). Embryos expressing WT Twist, or Twist carrying four or six C-terminal S to A mutations were cultured to blastula stages when the expressed proteins were immunoprecipitated and used as substrates in kinase assays with recombinant GSK-3β. WT Twist was robustly phosphorylated by GSK-3β in these assays, whereas the Twist C-terminus carrying 6SA mutations showed greatly diminished phosphorylation ( Fig. 5b ). Together, these data demonstrate that serines in the Twist C-terminus can serve as GSK-3β substrates in vitro . 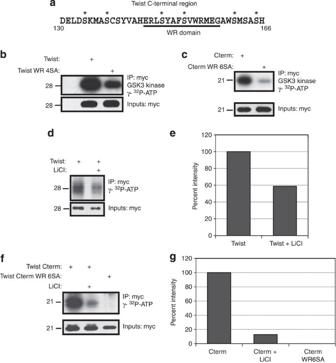Figure 5: Twist is a substrate for GSK-3β-mediated phosphorylation. (a) Amino-acid sequence of the Twist C terminus highlighting putative GSK3β target sites. The WR domain is underlined and the GSK3β consensus sequence serine residues (SxxxS) denoted by asterisks. (b)In vitrokinase assay showing GSK3β phosphorylation of full-length Twist. Myc-tagged Twist or Twist WR 4SA were IP from embryo lysates and used as substrates for recombinant GSK3β kinase (NEB) in the presence of [γ-32P]ATP. Kinase reactions were resolved by SDS–PAGE and visualized by autoradiography. (c)In vitrokinase assay showing GSK3β phosphorylation of the Twist. Myc-tagged WT Twist C terminus (Cterm) or Twist C terminus with all six serines mutated to alanine (Cterm WR 6SA) were immunoprecipitated from embryo lysates and used as substrates for recombinant GSK3β kinase (NEB) in the presence of [γ-32P]ATP. Kinase reactions were resolved by SDS–PAGE and visualized by autoradiography. (d) Inhibition of endogenous GSK3β by lithium chloride reduces Twist phosphorylation. Myc-tagged Twist was immunoprecipitated from injected embryo lysates, then incubated with [γ-32P]ATP and either untreated embryo lysates or lysates treated with 100 mM LiCl. Kinase reactions were resolved by SDS–PAGE and visualized by autoradiography. A reduction of phosphorylation is seen in LiCl-treated samples. (e) Graph quantifying phosphoimager percentage intensity readings of the samples in (d). (f) Inhibition of endogenous GSK3β by lithium chloride reduces phophoryation of the Twist C terminus (Twist Cterm). Myc-tagged Twist C-terminal isoforms (Twist Cterm or Twist Cterm 6SA) were immunoprecipitated from injected embryo lysates then incubated with [γ-32P]ATP and untreated embryo lysates or lysates treated with 100 mM LiCl. Kinase reactions were resolved by SDS–PAGE and visualized by autoradiography. (g) Graph quantifying phosphoimager percentage intensity readings of the samples in (f). Figure 5: Twist is a substrate for GSK-3β-mediated phosphorylation. ( a ) Amino-acid sequence of the Twist C terminus highlighting putative GSK3β target sites. The WR domain is underlined and the GSK3β consensus sequence serine residues (SxxxS) denoted by asterisks. ( b ) In vitro kinase assay showing GSK3β phosphorylation of full-length Twist. Myc-tagged Twist or Twist WR 4SA were IP from embryo lysates and used as substrates for recombinant GSK3β kinase (NEB) in the presence of [γ- 32 P]ATP. Kinase reactions were resolved by SDS–PAGE and visualized by autoradiography. ( c ) In vitro kinase assay showing GSK3β phosphorylation of the Twist. Myc-tagged WT Twist C terminus (Cterm) or Twist C terminus with all six serines mutated to alanine (Cterm WR 6SA) were immunoprecipitated from embryo lysates and used as substrates for recombinant GSK3β kinase (NEB) in the presence of [γ- 32 P]ATP. Kinase reactions were resolved by SDS–PAGE and visualized by autoradiography. ( d ) Inhibition of endogenous GSK3β by lithium chloride reduces Twist phosphorylation. Myc-tagged Twist was immunoprecipitated from injected embryo lysates, then incubated with [γ- 32 P]ATP and either untreated embryo lysates or lysates treated with 100 mM LiCl. Kinase reactions were resolved by SDS–PAGE and visualized by autoradiography. A reduction of phosphorylation is seen in LiCl-treated samples. ( e ) Graph quantifying phosphoimager percentage intensity readings of the samples in ( d ). ( f ) Inhibition of endogenous GSK3β by lithium chloride reduces phophoryation of the Twist C terminus (Twist Cterm). Myc-tagged Twist C-terminal isoforms (Twist Cterm or Twist Cterm 6SA) were immunoprecipitated from injected embryo lysates then incubated with [γ- 32 P]ATP and untreated embryo lysates or lysates treated with 100 mM LiCl. Kinase reactions were resolved by SDS–PAGE and visualized by autoradiography. ( g ) Graph quantifying phosphoimager percentage intensity readings of the samples in ( f ). Full size image To determine if Twist phosphorylation in embryo extracts requires GSK-3β activity, we asked if this phosphorylation was sensitive to LiCl, a known GSK-3β inhibitor [51] . For these assays, Twist was expressed in embryos, immunoprecipitated at stage 8 and immobilized immune complexes incubated with either untreated embryo lysates or lysates treated with 100 mM LiCl. Treatment with LiCl substantially reduced Twist phosphorylation ( Fig. 5d ). Moreover, the ability of LiCl treatment to inhibit phosphorylation of the Twist C-terminus was even more pronounced, and mutating the six serine residues in the C-terminus largely abolished phosphorylation ( Fig. 5f ). Together, these findings demonstrate that the Twist C-terminus is a bonafide GSK-3β substrate. Phosphorylated Twist inhibits Snail function We next examined the functional consequences of GSK-3β phosphorylation of the Twist C-terminus. We found that co-expression with GSK-3β renders Twist less stable ( Fig. 6a ), presumably owing to enhanced Ppa binding. Co-expression of Snail1 protected Twist from destabilization and preventing phosphorylation of the six C-terminal serines blocked association of Twist with Snail factors as well as destabilization ( Fig. 6b ). Interestingly, co-expression of Wnt8, which downregulates GSK-3β, led to decreased interaction between Twist and Snail2 ( Fig. 6c ). Collectively, our data suggested a model in which Twist binds to and inhibits the activity of Snail proteins, and GSK-3β-mediated phosphorylation of the Twist C-terminus serves to promote this function. We therefore hypothesized that unphosphorylated Twist would be a less effective Snail1/2 inhibitor. To test this hypothesis, embryos expressing Twist S148A or Twist S148D were examined for the effects on Snail2-mediated NC precursor formation. Snail2 expression induces ectopic NC formation in this assay, and while Twist S148D potently blocked its effects, Twist S148A did not ( Fig. 6d ). These findings support a model in which GSK-3β-mediated Twist phosphorylation regulates the functional inhibition of Snail family EMT regulatory factors. 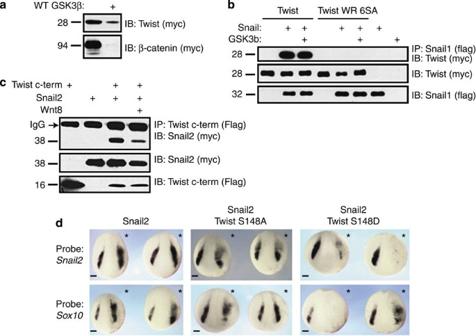Figure 6: Functional consequences of GSK3β phosphorylation. (a) Stability of Twist is decreased in the presence of GSK3β. Twist or β-catenin (as a positive control) were expressed in the presence or absence of GSK3β and collected at stage 8 to analyse Twist or β-catenin protein expression by western blot. Both proteins are destabilized by co-expressed GSK3β. (b) Co-IP of WT Twist or Twist WR 6SA by flag-tagged Snail1, in the presence or absence of co-expressed GSK3β. Immunoprecipitates were resolved by SDS–PAGE, and Snail1-bound Twist detected by α-Myc western blotting. Snail1 protects Twist from destabilization by GSK3β. Mutation of the 6 WR domain serines prevents interaction with Snail. (c) Western blot of co-IP showing that interaction between the Twist C-terminus and Snail2 is diminished when Wnt8 is co-expressed. (d)In situhybridization ofXenopusembryos expressing Snail2 in the presence or absence of Twist S148A or Twist S148D. Snail2 induces ectopic expression of neural crest markers Snail2andSox10, and Twist S148D potently interferes with this activity. Scale bars, 200 μm. IB, immunoblotting. * Denotes manipulated side of the embryo. Figure 6: Functional consequences of GSK3β phosphorylation. ( a ) Stability of Twist is decreased in the presence of GSK3β. Twist or β-catenin (as a positive control) were expressed in the presence or absence of GSK3β and collected at stage 8 to analyse Twist or β-catenin protein expression by western blot. Both proteins are destabilized by co-expressed GSK3β. ( b ) Co-IP of WT Twist or Twist WR 6SA by flag-tagged Snail1, in the presence or absence of co-expressed GSK3β. Immunoprecipitates were resolved by SDS–PAGE, and Snail1-bound Twist detected by α-Myc western blotting. Snail1 protects Twist from destabilization by GSK3β. Mutation of the 6 WR domain serines prevents interaction with Snail. ( c ) Western blot of co-IP showing that interaction between the Twist C-terminus and Snail2 is diminished when Wnt8 is co-expressed. ( d ) In situ hybridization of Xenopus embryos expressing Snail2 in the presence or absence of Twist S148A or Twist S148D. Snail2 induces ectopic expression of neural crest markers S nail2 and Sox10 , and Twist S148D potently interferes with this activity. Scale bars, 200 μm. IB, immunoblotting. * Denotes manipulated side of the embryo. Full size image A GRN describing the formation, migration and differentiation of NC cells is beginning to be delineated [17] , [18] , [19] . A central challenge to understanding complex developmental processes such as NC development on a systems level is determining how the function of proteins in the network are controlled individually and coordinately. This is particularly true for proteins, such as Twist, Snail1 and Snail2, which also function as core EMT regulatory factors. Twist is a particularly interesting component of this network. While Twist is expressed in cranial NC precursors in both Xenopus and zebrafish [15] , [52] , its early NC expression appears to have been lost in the mouse [16] , [53] , suggesting that Twist regulatory functions at these stages have been replaced by other factors in mammals. In the mouse, as in Xenopus , Twist is expressed in gastrula stage and presomitic mesoderm, and is also expressed in cranial and limb bud mesenchyme [16] , [53] . Heterozygous mutant Twist mice are viable but display abnormal craniofacial structures, while twist −/− mice have severe defects in cephalic neural tube closure and malformed branchial arches and facial primordium, showing that this protein is also essential for normal NC development in the mouse [16] , [53] . The co-expression of Twist and Snail1/2 in cranial NC precursors in Xenopus makes this an advantageous system to study functional interactions between these regulatory proteins, and such studies are important beyond the NC, because these factors also co-regulate other developmental events as well as tumour progression. We recently demonstrated that despite their structural diversity, Twist, a bHLH factor, and the zinc-finger transcriptional repressors Snail1/Snail2, are coordinately regulated. These factors, together with another core EMT factor Sip1, are targeted to the UPS by the same F-box protein, Ppa [36] . The functions of numerous developmental regulatory proteins are regulated, at least in part, by the threshold concentration of protein allowed to accumulate in cells. It is highly significant, however, that a common targeting mechanism has evolved to control the activity of a core group of functionally linked but structurally diverse factors. This suggests a need to control the activity of these factors as a unit as they direct complex developmental events and cellular behaviours. The uncovering of one shared mechanism for regulating the function of core EMT regulatory factors Twist and Snail1/2 raised the possibility that additional mechanisms exist for coordinately regulating these proteins. In the current study, we provide evidence for two further means by which Twist function can be regulated in concert with Snail1/Snail2. The observation that gain and loss of Twist function had similar consequences for some aspects of NC development suggested a possible functional dependence on protein–protein interaction, where proper stoichiometry is essential. Twist had been previously shown to maintain osteoblast precursors in an undifferentiated state via a mechanism involving binding and inhibiting Runx2 (ref. 33 ). This suggested that Twist might function, in part, by binding to and modulating the activity of other NC regulatory factors, and indeed we find strong DNA-independent interactions between Twist and the core EMT regulatory proteins Snail1/Snail2 (Slug). Interaction with Snail1/Snail2 did not interfere with the ability of Twist to bind DNA or dimerize (R Lander, unpublished data). Co-expression of Snail1 or Snail2 rendered Twist protein more stable, however, in part owing to competition for Ppa binding by Snail2 ( Fig. 4d ). Interaction between Twist and Snail1/2 is mediated by Twist’s C-terminal WR domain and by the C-terminal zinc fingers of Snail proteins, and diminishes recruitment of Snail2 to Ebox sequences in chromatin immunoprecipitation (ChIP) assays ( Supplementary Fig. S2 ). Interestingly, the Twist WR domain contains a serine residue previously shown to be important for Twist function (serine 152) that could represent a priming phosphorylation site for the GSK3-β regulation of serine 148. Two additional conserved SxxxS sites lie up and downstream of serine 148/152, and the clustering of such sites is a hallmark of canonical GSK-3β substrates, such as β-catenin and Ci 66,67 . We demonstrate using immune-complex kinase assays that GSK-3β can phosphorylate the Twist C terminus in a manner dependent on these sites. Moreover, phosphorylation of Twist by endogenous kinases in Xenopus embryo lysates displays strong sensitivity to LiCl, a known GSK-3β inhibitor, providing further evidence that Twist is a physiological target of GSK-3β phosphorylation. In the future, it will be important to investigate when and where Twist becomes phosphorylated by GSK-3β. Interestingly, mammalian Snail1 has also been shown to be a GSK-3β substrate, targeting it for beta-TrCP-mediated proteasomal degradation [54] , [55] , [56] . Although this regulation is not conserved in Snail2 or in amniote Snail1 proteins [34] , this nonetheless implicates GSK-3β phosphorylation as an additional regulatory mechanism common to these divergent core EMT factors. Multiple levels of shared regulation compellingly suggests that the activity of the core EMT factors must be controlled in concert for correct execution of their shared functions. Moreover, our findings suggest that an important role of phosphorylated Twist is to hold Snail1/2 activity in check, and that this function is regulated by GSK-3β. Further elucidation of the dynamic and coordinated regulation of these core EMT proteins as a functional unit will be an important area of future study. DNA constructs Epitope-tagged versions of all complementary DNAs were generated by amplifying the coding and inserting them into pCS2-MycC or pCS2-FlagC vectors. Xenopus Twist deletion mutants were generated using the following primers: Twist Nterm sense: 5′-ATGATGCAGGAA-3′, antisense: 5′-TCTCAAGGACGA-3′; Twist Cterm sense: 5′-ATGGCGAGCAGCACC-3′, antisense: 5′-GTGAGATGCAGA-3′; Twist ΔWR sense: 5′-ATGATGCAGGAA-3′, antisense: 5′-CACATAACTGCAGCTGGC-3′. The E12–WR domain fusion construct was generated by inserting the WR domain sequence (5′-GCCCATGAGAGGCTCAGCTATGCCTTCTCCGTGTGGAGGATGGAGGGAGC CTGGTCCATGTCTGCATCTCAC-3′) into the EcoRI site of Xenopus E12 in pCS2-MycC vector. All constructs were confirmed by sequencing. Embryological methods and cartilage staining All results shown are representative of at least three independent experiments. RNA for injection was produced in vitro from linearized plasmid templates using the Message Machine kit (Ambion). Embryos were injected at the 2-cell or 8-cell stage as noted and collected at the indicated stage. In situ hybridization was performed using digoxigenin-labelled RNA probes using the standard protocol [6] and developed using BM Purple substrate (Roche). Embryo images were collected on an Olympus dissecting microscope fitted with a × 10 objective and an Olympus QColor5 digital camera. Composite images were assembled using Adobe Photoshop. The Twist MO sequence is: 5′-CGGCACAATAAGGAGAAGGTCCCG -3′. For luciferase assays, firefly luciferase and Renilla constructs (DNA) were injected alone or in combination with Mitf and/or TwistΔWR RNA into both cells of a 2-cell Xenopus embryo. Embryos were cultured until stage 17, collected in 10-embryo sets and lysed in 500 μl of passive lysis buffer using the reporter assay system kit (Dual-Luciferase; Promega). The Dct -luciferase reporter contains the ~3.2-kb mouse Dct promoter. For cartilage staining, embryos were fixed in formaldehyde at stage 46 and stained overnight in 0.2% alcian blue/30% acetic acid in EtOH. Embryos were washed through a glycerol series into 80% glycerol/20% KOH before manual dissection of cartilages. Proliferation and TUNEL assays For phosphohistone H3 detection, Twist MO-injected or Twist messenger RNA-injected embryos were fixed in formaldehyde at stage 17 and processed for β-galactosidase activity. α-Phosphohistone H3 antibody (Upstate Biotechnology) was used at a concentration of 5 μg ml −1 ; α-rabbit IgG conjugated with alkaline phosphatase (Roche) was used at 1:1,000 and detected with BM Purple. For TUNEL assays, embryos injected with Twist MO or mRNA-encoding Twist were allowed to develop until stage 17. TUNEL staining was carried out as described previously [6] . Briefly, fixed embryos were rehydrated in PBT and washed in TdT buffer (Invitrogen) for 30 min. End labelling was carried out at room temperature overnight in TdT buffer containing 0.5 μM digoxigenin-dUTP (Roche) and 150 U ml −1 TdT (Invitrogen). Embryos were washed at 65 °C in PBS/1 mM EDTA and detection of the digoxigenin epitope was carried out as for in situ hybridization. IPs, western blots and stability assays For IPs, embryos were collected at stage 10, lysed in PBS+ 1% NP40 containing a protease inhibitor cocktail (Roche), and incubated with the indicated antibody (0.2 μg α-Myc (9E10, Santa Cruz) or 0.2 μg α-FlagM2 affinity purified (Sigma)) for 2 h on ice, followed by a 2 h incubation with protein A Sepharose beads. IPs were washed with RIPA buffer and resolved by SDS–polyacrylamide gel electrophoresis (PAGE). Immunoblotting was performed using α-Myc (1:2,000), affinity purified α-FlagM2 (1:3,000) or α-actin ((1:1,000), Sigma) antibody as indicated. Labelled proteins were detected using HRP-conjugated secondary antibodies and enhanced chemiluminescence (Amersham). Purification of GST proteins and GST pull-down assays GST proteins were expressed in BL21 stain of E. coli , sonicated and purified with glutathione-agarose (Sigma-Aldrich). Protein induction and bead attachment were verified by SDS–PAGE and Coomassie staining. Twist proteins were transcribed and translated in vitro using the quick coupled transcription/translation system (TNT) in the presence of [ 35 S]methionine. Eight percent of the reaction mixture was kept as the input. The remainder was incubated with glutathione bead-bound GST fusion proteins for 2 h at 4 °C in lysis buffer in a 500-μl volume. Glutathione-agarose was washed four times with RIPA buffer, and bound proteins were released by boiling in SDS sample buffer, analysed by SDS–PAGE and imaged using autoradiography. ChIP and quantitative PCR (qPCR) ChIP was performed with 50 embryos per IP and fold enrichment of transcription factor was quantified using SYBR green qPCR. Embryos were injected at 2-cell stage with RNA for myc-tagged Snail2 and/or Flag-tagged Twist at concentrations that correlate with endogenous levels. Expressed proteins levels were quantified using Odyssey licor scanner using infrared secondary antibody (Rockland #610-132-121). Embryos were harvested for ChIP at stage 17. IP for myc-tagged proteins were performed using anti-Myc epitope (Sigma #C3956) on Protein G magnetic beads (Dynabeads, Invitrogen #100-04D). qPCR was performed using primers for proximal promoters of Epidermal Keritin (Fwd: 5′-CCTGGAGCAAGGAGAGAGTG-3′; Rev: 5′-CGTAGCCTCAGGGTGTTTGT-3′) and, as a control, eEF1α (Fwd: 5′-TGCATGAAGCACAGCAGAAT-3′; Rev: 5′-CGGGTGAGGAAGAGAGGATT-3′) with SYBR Premix (Clontech #RR820W). Fold enrichment of Snail2 at the proximal promoters of Epidermal keratin and eEF1α was calculated using ΔΔC T method and represented as mean from three separate biological replicates with error bars representing s.e.m. In vitro and in vivo kinase assays For in vitro kinase assays, embryos were injected with RNA encoding Twist mutants (WR 6SA, WR 4SA and Cterm) at the 2-cell stage and collected at stage 8. Proteins were immunoprecipitated in the presence of 20 mM β-glycerol phosphate from embryo lysates as detailed above. Following RIPA washes, the immune complexes were washed two times in PBS and four times in 1 × GSK3 kinase buffer (NEB) and incubated with 1.5 μl 10 × GSK3 buffer, 0.5 μl 0.5 mM ATP (NEB), 0.5 μl 1M β-glycerol phosphate, 1 μl glycogen synthase kinase 3 (GSK-3) (NEB), 2 μl [γ- 32 P]ATP and 9.5 μl H 2 O for 20 min at 30 °C. Reactions were stopped with 1 μl of 5 mM EDTA. Immune complexes were then washed four times with PBS+20 mM EDTA, and resolved by SDS–PAGE and visualized by autoradiography. For in vivo kinase assays, Twist proteins were immunoprecipitated, and Twist-bound PAS beads were washed four times in X1 Extraction Buffer (XB) then incubated with 15 μl Xenopus embryo extract (see Method below), 0.5 μl [γ- 32 P]ATP, 100 mM LiCl (or H 2 O control) for 30 min at room temperature. Reactions were stopped with 1 μl of 5 mM EDTA and immune complexes were washed four times with PBS+20 mM EDTA, and samples were resolved by SDS–PAGE and visualized by autoradiography. Xenopus embryo extract preparation Extract preparation methods were adapted from Kim et al . [57] Fertilized Xenopus embryos were collected at stage 9 and washed four times with 1 × Extraction Buffer (XB) plus 20 mM β-glycerol phosphate and protease inhibitors. Embryos were incubated with 500 μl of 1 × XB (plus phosphatase/protease inhibitors and 10 μg ml −1 cytochalasin B) on ice for 3 min and then packed at a low speed (<100 g for 30 s). Excess liquid was removed and eggs were crushed at 21,000 g for 5 min at 4 °C. The clear, cytoplasmic middle layer was transferred to a new, chilled tube. Protease inhibitors and cytochalasin B were added to the extract. Four more rounds of centrifugation were then performed to obtain clear egg extracts. How to cite this article: Lander, R. et al . Interactions between Twist and other core epithelial–mesenchymal transition factors are controlled by GSK3-mediated phosphorylation. Nat. Commun. 4:1542 doi: 10.1038/ncomms2543 (2013).